Mechanism of outer membrane destabilization by global reduction of protein content 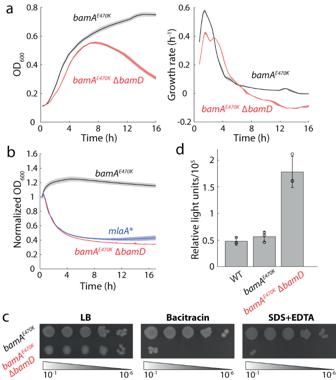Fig. 1: Deletion ofbamDleads to cell death during stationary phase and a highly permeable membrane. abamDdeletion leads to slower growth in log phase and a decrease in OD600in stationary phase compared with the parent strainbamAE470K. Left: OD600measurements starting from a diluted overnight culture.N= 3 biological replicates. Curves are mean values, and shaded regions represent 1 standard deviation. Right: corresponding growth rates as quantified bydln(OD)/dt.bΔbamDandmlaA* cells exhibited similar decreases in OD when transferred from log phase to the spent medium of wild-typeE. coliMC4100 cells, while the parent strain maintained a stable OD. All OD measurements were normalized to the value upon transfer to spent medium att= 0.N= 3 biological replicates. Curves are mean values, and shading represents 1 standard deviation.cΔbamDcells exhibited inhibited growth on plates with bacitracin or SDS-EDTA compared with LB plates, whereas growth of the parent strain was not affected by either treatment. Data are representative of three biological replicates.dΔbamDcells exhibited increased OM permeability compared with the parent strain as measured by the intake of fluorescent 1-N-phenyl-naphthylamine (NPN), normalized by OD600. Data are presented as mean values ± 1 standard deviation.N= 3 biological replicates. The outer membrane (OM) of Gram-negative bacteria such as Escherichia coli is an asymmetric bilayer with the glycolipid lipopolysaccharide (LPS) in the outer leaflet and glycerophospholipids in the inner. Nearly all integral OM proteins (OMPs) have a characteristic β-barrel fold and are assembled in the OM by the BAM complex, which contains one essential β-barrel protein (BamA), one essential lipoprotein (BamD), and three non-essential lipoproteins (BamBCE). A gain-of-function mutation in bamA enables survival in the absence of BamD, showing that the essential function of this protein is regulatory. Here, we demonstrate that the global reduction in OMPs caused by BamD loss weakens the OM, altering cell shape and causing OM rupture in spent medium. To fill the void created by OMP loss, phospholipids (PLs) flip into the outer leaflet. Under these conditions, mechanisms that remove PLs from the outer leaflet create tension between the OM leaflets, which contributes to membrane rupture. Rupture is prevented by suppressor mutations that release the tension by halting PL removal from the outer leaflet. However, these suppressors do not restore OM stiffness or normal cell shape, revealing a possible connection between OM stiffness and cell shape. Gram-negative bacteria such as Escherichia coli are protected from the environment by their cell envelope, which is made unique by the outer membrane (OM). The OM, an asymmetric bilayer with lipopolysaccharide (LPS) in the outer leaflet and glycerophospholipids (PLs) in the inner leaflet, functions as a selective permeability barrier, allowing passage of small hydrophilic compounds while excluding large and hydrophobic molecules [1] . An ordered network of outer membrane proteins (OMPs) with patches of LPS stabilized by electrostatic LPS-LPS and LPS-OMP interactions contribute to the mechanical strength of the cell [2] , [3] , [4] . Perturbation to this essential barrier can result in cell death. The integrity of the OM relies on proper localization of its multiple components. LPS is transported by the Lpt machinery, which is composed of seven proteins that form a trans-envelope bridge [5] . Asymmetry is then established by multiple mechanisms. First, the Mla system shuttles mislocalized PLs back to the inner membrane (IM) [6] . Second, the outer membrane phospholipase PldA breaks down mislocalized PLs and acts as a sensor of OM asymmetry [7] , [8] . While LPS transport and maintenance of OM asymmetry are well understood, PL transport to the OM remains poorly characterized. However, recent work indicates that PLs are transported from the IM to the inner leaflet of the OM by protein bridges using redundant AsmA-like proteins such as YhdP, TamB, and YdbH [9] , [10] , [11] , [12] . OMPs are typically β-barrel proteins that span the OM and are assembled by the β-barrel assembly machine (BAM) complex. The E. coli BAM complex is heteropentomeric, containing two essential proteins, BamA and BamD, and three non-essential proteins, BamB, BamC, and BamE. BamA, itself a β-barrel protein, catalyzes the folding of OMPs, while the lipoprotein BamD plays a regulatory and substrate quality control role in OMP assembly [13] , [14] . Previous work identified an allele of bamA , bamA E470K , that is viable in the absence of bamD [14] . Deletion of bamD in the bamA E470K background results in increased OM permeability [14] , but the structural changes underlying this phenotype are not well understood. In this work, we investigate the consequences of bamD deletion on the structural integrity of the OM and on cell shape. bamD deletion resulted in a highly inefficient BAM complex, leading to decreased OMP levels and mislocalization of PLs to the outer leaflet of the OM [14] . We show that these structural changes alter growth rate and cell shape and cause a striking cell death phenotype, precipitated by rupture of the OM in spent medium or under oscillatory hyperosmotic shocks. Suppressor analysis suggested that mechanisms that remove PLs from the OM outer leaflet under protein-depleted conditions create interleaflet tension that destabilizes the OM. Relieving this tension through suppressor mutations rescued cell death, but altered cell shape and OM mechanical stiffness remained compromised, emphasizing the central role of OM proteins and OM stiffness in cellular morphogenesis and integrity. Deletion of bamD decreases fitness in stationary phase and causes OM permeability defects A previous study showed that bamA E470K cells can tolerate deletion of bamD [14] . Given the otherwise essential role of bamD , we sought to further characterize the effects of bamD deletion on cellular physiology. As observed previously, overnight cultures of a bamA E470K ∆ bamD strain (hereafter, ∆ bamD ) exhibited lower optical density (OD) than the parent bamA E470K strain [14] , and ∆ bamD cultures exhibited lower maximum growth rate and pronounced lysis during stationary phase compared with the parent (Fig. 1a ). To further interrogate the stationary phase lysis of ∆ bamD cultures, we resuspended log-phase cells in LB supernatant collected by filtering the cells from an overnight wild-type culture (“spent medium”), which lacks the nutrients needed to support growth and rapidly transitions cells into stationary phase. This spent medium assay was used previously to probe membrane integrity in cells with the mlaA* allele [15] , which disrupts OM lipid homeostasis. Δ bamD and MC4100 mlaA* cells exhibited nearly identical lysis dynamics upon transitioning to spent medium, while the OD of the parent remained high (Fig. 1b ). Since spent LB lacks the Mg 2+ necessary to stabilize LPS-LPS interactions, we reasoned that the weakened OM of the Δ bamD mutant was not able to withstand the additional stress. Indeed, when we supplemented spent LB with Mg 2+ , lysis was abolished (Fig. S 1 ). Fig. 1: Deletion of bamD leads to cell death during stationary phase and a highly permeable membrane. a bamD deletion leads to slower growth in log phase and a decrease in OD 600 in stationary phase compared with the parent strain bamA E470K . Left: OD 600 measurements starting from a diluted overnight culture. N = 3 biological replicates. Curves are mean values, and shaded regions represent 1 standard deviation. Right: corresponding growth rates as quantified by d ln(OD)/ dt . b Δ bamD and mlaA * cells exhibited similar decreases in OD when transferred from log phase to the spent medium of wild-type E. coli MC4100 cells, while the parent strain maintained a stable OD. All OD measurements were normalized to the value upon transfer to spent medium at t = 0. N = 3 biological replicates. Curves are mean values, and shading represents 1 standard deviation. c Δ bamD cells exhibited inhibited growth on plates with bacitracin or SDS-EDTA compared with LB plates, whereas growth of the parent strain was not affected by either treatment. Data are representative of three biological replicates. d Δ bamD cells exhibited increased OM permeability compared with the parent strain as measured by the intake of fluorescent 1-N-phenyl-naphthylamine (NPN), normalized by OD 600 . Data are presented as mean values ± 1 standard deviation. N = 3 biological replicates. Full size image Δ bamD colonies were very mucoid, suggesting that the Rcs stress response is activated due to perturbations to the OM. To probe the integrity of the OM, we plated parent and Δ bamD cells on LB and LB supplemented with bacitracin, a large hydrophilic peptide antibiotic that is typically excluded from E. coli cells [16] , or SDS-EDTA. Δ bamD cells were unable to grow in the presence of bacitracin or SDS-EDTA (Fig. 1c ). To further test OM permeability, we quantified uptake of fluorescent 1-N-phenyl-naphthylamine (NPN) [17] . After 20 min, wild-type MC4100 and bamA E470K cells displayed much lower uptake than Δ bamD cells (Fig. 1d ), indicating that bamD deletion generally increased OM permeability. Together, these results indicate that bamD deletion dramatically alters the OM. bamD deletion reduces growth rate and disrupts cell shape We noted that deletion of bamD decreased the maximal growth rate in exponential phase (Fig. 1a ), and sought to characterize the effect of bamD deletion on cell shape and single-cell growth dynamics. Using time-lapse imaging, we tracked single cells from log-phase cultures on an LB agarose pad and quantified single-cell growth rates (Fig. 2a, b ). ∆ bamD cells exhibited disrupted shapes, usually featuring more nonuniform cell width along the cell body and greater elongation compared with the parent (Fig. 2a , Movie S1 , S2 ), indicating disrupted shape regulation. The average instantaneous growth rate of ∆ bamD cells was significantly lower than that of wild-type cells even when controlling for similar cell shape (Fig. 2b ), consistent with population growth measurements (Fig. 1a ). Moreover, instantaneous growth rate decreased as the cell-width coefficient of variation increased (Fig. 2b ), suggesting that deletion of bamD causes a metabolic burden linked to envelope disruption. Some cells eventually lysed (Fig. 2a , arrows), signifying weakening of the cell envelope. Additionally, we quantified the morphology of two other BAM complex mutants: bamA101 , a transposon insertion in the bamA promoter that decreases BamA levels by >90%, and deletion of bamB , which encodes a nonessential BAM complex lipoprotein. We selected ∆ bamB because this mutant has greater permeability defects than ∆ bamC or ∆ bamE mutants [18] , [19] , [20] . The bamA101 and ∆ bamB mutants showed disrupted regulation of cell width compared to bamA E470K (Fig. S 2a ). Thus, disrupting the BAM complex has global effects on cell morphology and growth. Fig. 2: ∆ bamD cells exhibit defects in growth rate and cell shape, and the outer membrane ruptures before the inner membrane in spent medium. a As compared with the parent strain, Δ bamD cells exhibit more variation in cell width along the cell body as well as lysis (red arrows). Shown are time-lapse images of log-phase cells on an agarose pad with LB. Scale bar: 5 µm. b Δ bamD cells had lower instantaneous growth rates ( d ln A / dt , where A is cell area; top) compared with the parent strain. Shown are cells grouped based on the degree of cell shape defect (bottom), as quantified by the coefficient of variation of width along the cell body (Methods). Error bars represent 25th and 75th percentiles. Example cell contours for each grouping are shown under the corresponding bar plots. The number of cells in each group is shown on the barplot. Two-sample Kolmogorov-Smirnov test; **: p < 0.01, ***: p < 0.001. 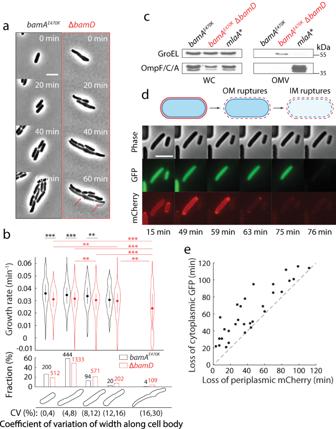Fig. 2: ∆bamDcells exhibit defects in growth rate and cell shape, and the outer membrane ruptures before the inner membrane in spent medium. aAs compared with the parent strain, ΔbamDcells exhibit more variation in cell width along the cell body as well as lysis (red arrows). Shown are time-lapse images of log-phase cells on an agarose pad with LB. Scale bar: 5 µm.bΔbamDcells had lower instantaneous growth rates (dlnA/dt, whereAis cell area; top) compared with the parent strain. Shown are cells grouped based on the degree of cell shape defect (bottom), as quantified by the coefficient of variation of width along the cell body (Methods). Error bars represent 25th and 75th percentiles. Example cell contours for each grouping are shown under the corresponding bar plots. The number of cells in each group is shown on the barplot. Two-sample Kolmogorov-Smirnov test; **:p< 0.01, ***:p< 0.001. Exactp-values are included in Supplementary Table2.cImmunoblots of OM porins in the whole cell (WC) or OM vesicles (OMVs) ofbamAE470K, ΔbamD, andmlaA*cultures, compared to the level of the intracellular protein GroEL used as a control. Deletion ofbamDdoes not induce OMV production, by contrast to themlaA* allele. Data are representative of three biological replicates.dIn a ∆bamDcell shifted from log-phase growth in LB to spent LB, the OM ruptures before the IM. Shown are time-lapse images of ∆bamDcells expressing cytoplasmic GFP and periplasmic mCherry incubated in a microfluidic flow cell (Methods). The longer cell on the left maintained cytoplasmic GFP for >15 min after periplasmic mCherry was lost. Scale bar: 5 µm.eFor all cells measured as in (d), periplasmic mCherry was lost earlier or at the same time as cytoplasmic GFP in ΔbamDcells shifted from log phase growth in LB to spent LB.n= 30 cells. Exact p -values are included in Supplementary Table 2 . c Immunoblots of OM porins in the whole cell (WC) or OM vesicles (OMVs) of bamA E470K , Δ bamD , and mlaA* cultures, compared to the level of the intracellular protein GroEL used as a control. Deletion of bamD does not induce OMV production, by contrast to the mlaA * allele. Data are representative of three biological replicates. d In a ∆ bamD cell shifted from log-phase growth in LB to spent LB, the OM ruptures before the IM. Shown are time-lapse images of ∆ bamD cells expressing cytoplasmic GFP and periplasmic mCherry incubated in a microfluidic flow cell (Methods). The longer cell on the left maintained cytoplasmic GFP for >15 min after periplasmic mCherry was lost. Scale bar: 5 µm. e For all cells measured as in ( d ), periplasmic mCherry was lost earlier or at the same time as cytoplasmic GFP in Δ bamD cells shifted from log phase growth in LB to spent LB. n = 30 cells. Full size image The OM ruptures prior to the IM in ∆ bamD cells when transitioned to spent medium Based on the similarity of lysis dynamics upon starvation in mlaA * cells and ∆ bamD cells (Fig. 1b) , we hypothesized based on our previous findings [15] that bamD deletion leads to loss of outer membrane material via vesiculation. To test this hypothesis, we collected outer membrane vesicles (OMVs) from exponentially growing cells (Methods). While we were able to easily harvest OMVs from mlaA * cells, preparations from parent or Δ bamD cells displayed no detectable OM proteins (Fig. 2c ). Instead, in Δ bamD cells we detected the cytoplasmic protein GroEL, suggesting leakiness due to cell rupture during the centrifugation used for OMV harvest. To identify the mechanism by which Δ bamD cells lyse in spent medium, we used a microfluidic flow cell to rapidly transition log-phase cells to spent medium (Methods). Motivated by our previous study in which we showed that the IM ruptures before the OM in mlaA* cells [11] , we utilized a ∆ bamD strain that constitutively expresses cytoplasmic GFP and periplasmic mCherry (Table S1 ). Time-lapse imaging revealed that periplasmic mCherry fluorescence was always lost prior to (Fig. 2d ) or coincident with the loss of cytoplasmic GFP (Fig. 2e ), indicating that the OM ruptured before the IM. Together, these data indicate that a severely destabilized OM is the direct cause of ∆ bamD cell lysis in stationary phase. OM composition is altered by bamD deletion To further interrogate the lysis phenotype, we collected cell lysate from cells grown at 37 °C in log phase (Methods) and measured the abundance of OM components such as the major OM porins (Fig. 3a , lane 1 and 2; Fig. 3b , lane 1 and 2) and LPS (Fig. 3b , lane 1 and 2). Deletion of bamD dramatically decreased levels of OM porins, including the essential BamA and LptD. By contrast, LPS levels were relatively unaffected by bamD deletion even though LptD levels were decreased (Fig. 3b , lane 1 and 2). Taken together, these results indicate that the OM of Δ bamD cells is highly lacking in proteins, and that lysis is not due to membrane loss but instead due to altered OM composition. Fig. 3: OM lysis is not due to loss of material but instead due to alteration in membrane composition. a bamD deletion reduces levels of OM proteins. Shown are immunoblots of major OM proteins in cell lysates of bamA E470K , Δ bamD , and suppressor mutants of Δ bamD from log-phase cultures. Data are representative of three biological replicates. b Although deletion of bamD reduces levels of the LPS transport protein LptD, LPS levels are unaffected. Shown are immunoblots of LptD, GroEL (as a control), and LPS in cell lysates of bamA E470K , Δ bamD , and suppressor mutants of Δ bamD from log-phase cultures. Data are representative of three biological replicates. c The decrease in OD in stationary phase (left) or upon transition from log-phase growth to spent LB (right, transition occurs at t = 0) in ∆ bamD cells is partially rescued by deletion of pldA and fully rescued by deletion of pldA and mlaA . N = 3 biological replicates. Curves are mean values, and shading represents 1 standard deviation. d Cell lysis in spent LB is partially rescued by deletion of pldA and almost fully rescued by deletion of pldA and mlaA , in agreement with the population-level measurements in ( c ). Shown are quantifications of the fraction of viable cells as determined from time-lapse images (Methods). n > 100 cells for each strain. e Suppressors do not rescue the permeability defect of ∆ bamD cells. Shown is quantification of the intake of fluorescent 1-N-phenyl-naphthylamine (NPN) in bamA E470K , Δ bamD , and suppressor mutants. Data are presented as mean values ± 1 standard deviation. N = 3 biological replicates. Relative light units = fluorescence/OD 600 . Full size image Mutants that increase PL levels in the OM outer leaflet suppress lysis due to bamD deletion Efforts to isolate spontaneous suppressors of ∆ bamD lysis were unsuccessful, hence we attempted to identify rescue conditions for growth and decreased lysis through strategic genetic manipulation of the OM. In previous work, we identified the OM outer leaflet phospholipase PldA as a potent suppressor of mlaA * lysis [15] . Deletion of pldA from Δ bamD cells slowed down lysis kinetics in both stationary phase and the spent medium assay, and moderately improved the initial growth dynamics (Fig. 3c ). We reasoned that since ∆ bamD cells are lacking in many proteins that typically make up a large fraction of the OM, deletion of pldA allowed the cells to retain more PLs to fill the voids. Thus, by analogy with Acinetobacter baumannii mutants that lack LPS, we reasoned that other mutations that allow PLs to accumulate in the OM outer leaflet might also act as suppressors of Δ bamD lysis [21] , [22] . As shown in previous studies, inhibiting the Mla transport system and deleting pldA increases PL levels in the OM outer leaflet by ~25-fold and drastically changes OM physiology [2] , [6] . We found that deletion of mlaA from Δ bamD cells was not sufficient to rescue lysis (Fig. 3c ). Nonetheless, lysis was virtually abolished in Δ bamD Δ pldA Δ mlaA cells in both stationary phase and spent medium (Fig. 3c ). Single-cell lysis dynamics of the suppressors Δ bamD Δ pldA , Δ bamD Δ mlaA , and Δ bamD Δ pldA Δ mlaA upon exposure to spent medium (Fig. 3d ) closely mimicked population-level measurements (Fig. 3c ). The lpxC101 allele decreases lipid A biosynthesis [23] , [24] and frees up precursors for PL synthesis, leading to increased levels of PLs in the outer leaflet of the OM [25] . Introduction of lpxC101 to ∆ bamD cells improved growth dynamics and ameliorated lysis similar to the deletion of mlaA (Fig. S 3a ). Moreover, the combination of lpxC101 with Δ bamD Δ pldA restored growth dynamics and final yield to approximately that of the bamA E470K parent and lysis in stationary phase and the spent medium assay was completely abolished (Fig. S 3a, b ). Δ bamD lpxC101 Δ mlaA cells still showed lysis in spend medium, suggesting that PldA activity is detrimental in the Δ bamD background (Fig. S 3c ). To investigate the basis for rescue, we first tested whether the Bam complex was functioning more efficiently in the suppressor backgrounds. The Δ bamD Δ mlaA Δ pldA and Δ bamD lpxC101 Δ pldA suppressors of lysis did not restore OMP levels to that of wild type, nor did any of the other single mutants (Fig. 3b ). Moreover, levels of oxidized or reduced LptD showed a similar pattern in all mutants, and LPS levels were only reduced in strains with the lpxC101 allele (Fig. 3b ). As noted above, the ∆ bamD colonies are mucoid, indicating production of the colanic acid capsule. Since E. coli K-12 strains lack an O-antigen, the O-antigen ligase attaches colanic acid to LPS, producing a larger, modified form of LPS. This modification did not affect the lysis phenotype, as disruption of the upstream Rcs pathway did not reduce the degree of lysis (Fig. S 4 ). The Δ bamD Δ mlaA Δ pldA and Δ bamD lpxC101 Δ pldA suppressor mutants had a similar increase in permeability in our NPN assay relative to the parent (Fig. 3e ). Collectively, these data suggest that prevention of lysis depends on PL levels in the OM outer leaflet, and not restoration of protein networks or LPS modification. Populating the OM outer leaflet with PLs does not restore cell shape or viability under large osmotic shocks One of the essential functions of the bacterial OM is to provide mechanical integrity for withstanding forces from inside and outside of the cell [3] , [26] . The stiffness of the OM is largely determined by molecular interactions among outer membrane components including proteins and LPS molecules and between the OM and the cell wall [2] , [3] , [4] . Based on the altered OM composition of the Δ bamD strain and its suppressors (Fig. 3a, b ), we hypothesized that a reduction in OM protein levels or increased PLs would affect the stiffness of the OM. To quantify sensitivity to mechanical perturbations, we performed oscillatory hyperosmotic shock assays in a microfluidic flow cell (Methods) [3] , [27] . Δ bamD cells exhibited a drastic reduction in viability compared to the parent strain (Fig. 4a , Movie S3 ). While Δ bamD ∆ mlaA Δ pldA cells did not exhibit lysis in spent medium (Fig. 3c, d ), they were still more sensitive to large osmotic shocks than the parent strain (Fig. 4a ). Fig. 4: Replacement of proteins with PLs does not restore cell shape or OM stiffness. a Lysis due to oscillatory hyperosmotic shocks (cycles of 1 min in LB and 1 min in LB + 400 mM sorbitol; Methods) is partially rescued by deletion of both pldA and mlaA . Shown are measurements of the fraction of viable cells from time-lapse images in a microfluidic flow cell. n = 60 for bamA E470K ; n > 100 cells for all other strains. b Δ bamD and Δ bamD Δ pldA Δ mlaA cells have lower OM stiffness than the parent strain. Shown are measurements of cell wall length contraction from the turgid state to plasmolyzed state after addition of 1 M sorbitol (ε 12 ), from the plasmolyzed state to lysed state after addition of detergent (ε 23 ), and from the turgid state to the lysed state (ε 13 ) (Methods). ε 12 and ε 23 are higher and lower, respectively, in Δ bamD and Δ bamD Δ pldA Δ mlaA compared with the parent strain, suggesting that the OM in the two mutants is not as able to resist contraction upon turgor release. Data are presented as mean values ± 1 standard deviation. Sample sizes: n = 17 for bamA E470K , n = 24 for Δ bamD (plus 6 cells for ε 12 only), n = 20 for Δ bamD Δ pldA Δ mlaA . c The OM rest length is similar to that of the turgid cell in bamA E470K , Δ bamD , and Δ bamD Δ pldA Δ mlaA cells, indicating that the OM of all strains have a similar amount of material. Shown is the ratio of the OM size of a spheroplast compared to the turgid OM area (Methods). In all three strains, the OM rest length is substantially larger than a cell after plasmolysis (ratio of OM length after plasmolysis to the turgid length is shown as grey dashed lines). N = 1 biological replicate. Data are presented as mean values ± 1 standard deviation. Sample sizes: n = 13 for bamA E470K , n = 11 for Δ bamD , n = 20 for Δ bamD Δ pldA Δ mlaA . d Cell shape defects due to bamD deletion are not rescued in the suppressor strains Δ bamD Δ pldA , Δ bamD Δ mlaA , and Δ bamD Δ pldA Δ mlaA . All three strains exhibited higher coefficient of variation in cell width along the cell body compared to the parent. Lines are colored by strain as in ( a ). n > 200 cells for each strain. Insets: cells were imaged during log-phase growth in a microfluidic flow cell. Scale bar: 10 µm. Full size image Previously, we quantified the stiffness of the OM in various Gram-negative bacteria using a plasmolysis/lysis assay in which cells were exposed first to a large hyperosmotic shock to remove turgor pressure and then a detergent or EDTA to lyse the cells (Methods) [3] . Consistent with our previous findings, cell length of the parent strain decreased by ~12% upon plasmolysis and then by a further ~11% upon lysis (Fig. 4b ), indicating that compression of the stiff outer membrane was holding the cell wall in an extended state during plasmolysis. By contrast, Δ bamD and Δ bamD Δ pldA Δ mlaA cells shrank by ~30% upon plasmolysis and exhibited very little further contraction upon lysis (Fig. 4b ), suggesting that the OM in these strains is much weaker than the parent strain. Interestingly, the stiffness of the OM in the bamA101 and Δ bamB mutants was similar to that of bamA E470K cells, as indicated by the comparable cell length contraction upon plasmolysis and subsequent cell lysis (Fig. S 2b ). Similar to a spring, contraction upon plasmolysis is determined by a combination of the stiffness and rest length (amount of material) of the OM. We previously showed in wild-type cells that the OM rest length is similar to the length of the turgid cell [3] , indicating that there is little stress in the OM during steady-state growth. Mimicking these findings, we found that OM rest length in bamA E470K , ∆ bamD , and ∆ bamD ∆ pldA ∆ mlaA cells was similar to the length of the turgid cell and significantly larger than the plasmolyzed length, which is ~75% of the turgid cell length (Fig. 4c , Methods). In other words, even though the OM of ∆ bamD cells lacks OMPs, the amount of material in the OM is not substantially lower than in wild-type cells. By assuming that the OM rest length is equivalent to the turgid length, we estimated the mean OM stiffness (Methods) to be ~90% and ~75% lower in ∆ bamD and ∆ bamD ∆ pldA ∆ mlaA cells, respectively, compared with bamA E470K cells. Moreover, exponentially growing ∆ bamD Δ pldA , ∆ bamD ∆ mlaA , and ∆ bamD ∆ mlaA Δ pldA cells all exhibited disrupted cell shapes (Fig. 4d ), similar to ∆ bamD cells (Fig. 2a ). Taken together, we infer that reduction in the levels of OM proteins mechanically destabilized the OM, and increasing the levels of PLs by deleting pldA and mlaA does not restore mechanical integrity. Our results demonstrate that a global decrease in OMP levels resulting from lack of BamD in the BAM complex compromises cell viability and shape. The destabilized OM ruptures during stationary phase due to increased tension and has significantly decreased stiffness with which to withstand mechanical stress. As observed previously with A. baumannii [21] , [22] , to populate voids in the OM caused by the lack of OM components in E. coli ∆ bamD cells, PLs flip from the inner leaflet of the OM to the outer leaflet. In the case of A. baumannii , the OM component lacking was LPS, while E. coli ∆ bamD it was OMPs. In both organisms, PldA and Mla pathway activityes are detrimental, and both activities must be removed to relieve the defects. It is likely that the OMP defect is more severe than the LPS defect. A. baumannii strains lacking LPS exhibit growth defects [22] , while in E. coli ∆ bamD , the OMP defects both slow growth and cause cell lysis in spent media. In vitro studies with purified PldA suggest that the enzyme binds diacyl compounds three to five times better than monoacyl compounds, demonstrating a preference for PLs [28] . Thus, in an envelope that has an abundance of PLs, the majority of PldA activity may be generating lyso-phospholipids rather than fully breaking down the PLs. In turn, lyso-phospholipids have been implicated in changes to local membrane properties and in modification of embedded protein function [29] , [30] . We suggest that the decreased production of these lyso-phospholipids explains why removing PldA has a greater effect on cellular viability of the ∆ bamD mutant than does removal of the Mla transport system. Gram-negative bacteria possess several mechanisms for maintaining lipid asymmetry in the OM and as such, there is likely no mechanism for flipping PLs from the inner leaflet to the outer leaflet; such an activity would be counterproductive. In strains where PLs are needed in the outer leaflet to fill the void created by the absence of one of the major OM components, uncatalyzed PL flipping happens slowly and the resulting imbalance in material content creates tension between the membrane leaflets (Fig. 5 ). To make matters worse, PLs are further limited in the outer leaflet via rapid degradation by PldA and the activity of the Mla transport system (Fig. 5 ). We hypothesize that by populating the outer leaflet with PLs, interleaflet membrane tension is decreased, growth defects are ameliorated, and OMP-depleted E. coli cells can survive in nutrient- and cation-depleted spent LB (Fig. 5 ). Interestingly, while the growth defects and lysis can be suppressed in the ∆ pldA ∆ mlaA double mutant, the suppressor mutations do not restore mechanical integrity, the OM permeability barrier, or cell shape (Fig. 5 ). Fig. 5: Model of OM destabilization by the severe reduction in protein content due to bamD deletion. When ∆ bamD cells are transferred from log-phase growth to spent LB or exposed to oscillatory osmotic shocks, they exhibit much higher rates of cell lysis than the parent bamA E470K strain, due to a reduction in OMP levels and consequent decrease in OM stiffness. Deletion of mlaA and pldA increases the amount of PLs in the outer leaflet of the OM, which relieves interleaflet tension and prevents lysis in spent medium. However, the ∆ bamD ∆ mlaA ∆ pldA mutant exhibits only partial rescue of lysis under oscillatory osmotic shock and OM stiffness remains low. Full size image Together, our data combined with the previous studies of LPS- or lipooligosaccharide (LOS)-deficient A. baumannii suggest that the intact, ordered OMP network stabilized by LPS-LPS and LPS-protein interactions [2] , [3] , [4] are required to form a stiff OM. Our previous study implicated both LPS and OMPs as partial contributors to OM stiffness [3] . The reduction of OMP levels in ∆ bamD cells destroys the ordered OMP network and LPS presumably forms disconnected islands, leading to almost complete loss of OM stiffness. Proposed mechanisms of cell shape determination in bacteria tend to focus on the peptidoglycan cell wall due to its solid-like structure and ability to maintain its shape in the absence of other components [31] . However, our suppressor mutants imply the existence of a connection between OM stiffness and cell shape regulation, with a stiff OM mechanically restraining cell width fluctuations during growth and preventing the development of irregular cell shapes. PBP1A glycosyltransferase activity is lethal for LOS-deficient A. baumannii strains, suggesting that it is PBP1A activity that is affected by OM stiffness, leading to the observed irregular cell shapes in ∆ bamD cells [32] . The ability to perturb specific components of the complex OM composition, in this case OMPs through bamD deletion, thus provides insight into a distinct physiological state in which new mechanisms of cell envelope regulation can be revealed. Bacterial strains and growth conditions Strains, plasmids, and oligonucleotides are listed in Table S1 . Strains were grown in lysogeny broth (LB) supplemented with 25 mg/L kanamycin, 25 mg/L ampicillin, or 25 mg/L tetracycline when appropriate. Strains were maintained at 30 °C to decrease the frequency of lysis, while experimental data were acquired at 37 °C. bamA E470K was generated at the native bamA locus through recombineering using Collinsella stercoris phage RecT (CspRecT) as described previously [33] . All other chromosomal mutations were constructed using generalized transduction [34] . Deletions originated from the Keio collection [35] . Kanamycin resistance cassettes were excised using the FLP recombinase as described previously [36] . Growth curves Overnight cultures were diluted 1:100 in fresh LB and grown at 30 °C for 2 h. Optical density was measured, and cells were diluted to OD 600 = 0.05 in 500 mL of LB in a 24-well plate (CytoOne, USA Scientific, Cat. #CC7682-7524). The plate was covered with a Breathe-Easy gas-permeable membrane (Sigma-Aldrich, Cat. #Z380059) and grown overnight in a Synergy H1 microplate reader (BioTek) at 37 °C with continuous orbital shaking at 559 cpm frequency. OD 600 was measured every 15 min for 18 h. Lysis curves To make spent media, the wild-type MC4100 strain was grown in LB medium overnight, followed by centrifugation and filtration through a 0.2-µm filter to create cell-free spent medium. Early exponential phase cells (OD 600 = 0.6–0.8) were concentrated to OD 600 = 1 via centrifugation. Supernatant was discarded and the cell pellet was resuspended in 1 mL of spent medium, transferred to a 24-well plate (CytoOne, USA Scientific, Cat. #CC7682-7524), and covered with a Breathe-Easy gas-permeable membrane (Sigma-Aldrich, Cat. #Z380059). Lysis was monitored by decrease in optical density in a Synergy H1 microplate reader (BioTek) at 37 °C with continuous orbital shaking at 559 cpm frequency. OD 600 was measured every 15 min for 18 h. Efficiency of plating assay Exponential phase cultures were normalized to OD 600 = 1 and serially diluted 10-fold in LB medium in a 96-well plate. Cells were spotted using a 96-well replica plater onto the indicated media and incubated at 37 °C overnight. 1-N-phenylnapthylamine (NPN) uptake assay The NPN assay was performed as described previously [17] . Overnight cultures were diluted and grown to OD 600 = 0.6-0.8, and then normalized to OD 600 = 0.5. Cells were washed and resuspended in 5 mM HEPES buffer (pH 7.2). Two hundred microliters of cells were aliquoted into a clear-bottom black-well plate (Corning Incorporated, Cat. #3603). NPN was added at a final concentration of 10 μM. The plate was sealed with a Breathe-Easy gas-permeable membrane (Sigma-Aldrich, Cat. #Z380059) and incubated in a Synergy H1 microplate reader (BioTek). Fluorescence (excitation 350 nm, emission 420 nm) was measured after 20 min of incubation. Immunoblot analyses Exponentially growing cells were normalized to OD 600 = 1 and harvested by centrifugation. Cell pellets were resuspended in lysis buffer (25 mM Tris [pH 6.8], 1% SDS) and boiled for 5 min, followed by centrifugation. Supernatant was collected and protein concentration was measured using the Pierce BCA protein assay kit (ThermoFisher, Cat. #23225). Ten micrograms of protein were diluted in 4X Laemelli sample buffer (Bio-Rad, Cat. #1610747) supplemented with β-mercaptoethanol (except LptD-oxidized samples, for which β-mercaptoethanol was left out), and boiled for 10 min. Samples were loaded on an 8% (LptD samples) or 10% (all others) SDS-polyacrylamide gel, and electrophoresed. Proteins were transferred onto a nitrocellulose membrane using the Trans-Blot Turbo Transfer system (BioRad, Cat. #1704150) and membranes were blocked for 1 h in 5% milk at room temperature. Immunoblotting was performed using polyclonal antisera against BamA (1:25,000 dilution), OmpF/C/A (1:25,000 dilution), LamB/MBP (1:12,500 dilution), or monoclonal antibody recognizing GroEL (1:50,000, Sigma-Aldrich, Cat. #G6532) or FLAG (1:5000 dilution, Sigma-Aldrich, Cat. #F3165), followed by secondary antibodies goat anti-rabbit IgG horseradish peroxidase (1:10,000 dilution, Sigma-Aldrich, Cat. #12-348) or goat anti-mouse IgG horseradish peroxidase (1:10,000 dilution, BioRad, Cat. #1706516). LPS analysis LPS levels were analyzed as previously described [8] . Cells were grown to exponential phase and an OD 600 = 1 culture was obtained by centrifugation. The cell pellet was washed with PBS and resuspended in 100 μL of 1X NuPAGE LDS sample buffer (ThermoFisher, Cat. #NP0007) supplemented with 4% β-mercaptoethanol. Samples were boiled for 10 min and 2 μL of 20 mg/ml proteinase K (New England Biolabs, Cat. #P8107S) were added. Samples were incubated at 55 °C for 16 h, followed by inactivation by boiling for 5 min. Lysates were loaded onto a 4–12% NuPAGE Bis-Tris gradient gel (ThermoFisher, Cat. #NP0322BOX) and resolved by SDS-PAGE. Gels were stained with Pro-Q Emerald 300 Lipopolysaccharide Gel Stain kit (ThermoFisher, Cat. #P20495) using manufacturer’s instructions. LPS bands were visualized by UV transillumination. Fractionation of OM vesicles (OMVs) OMVs were collected as described previously [8] . Briefly, overnight cultures were diluted 1:100 into fresh LB and grown to OD 600 = 0.6-0.8. To collect whole-cell lysate controls, an OD 600 = 1 culture was obtained by centrifugation, resuspended in 50 µL of 2X Laemmli buffer (BioRad, Cat. #1610747) with 10% β-mercaptoethanol (MilliporeSigma, Cat. #M3148), and boiled for 10 min. To collect OMVs, an OD 600 = 3 culture was obtained by centrifugation. Supernatants were collected and adjusted to equal volume with fresh LB. Supernatants were filtered through a 0.2-μm filter (MilliporeSigma, Cat. #SLGPR33RB) and then through an Amicon Ultra-15 centrifugal filter with 100 kDa molecular weight cutoff (MilliporeSigma, Cat. #UFC9100) to isolate and concentrate OMVs. Centrifuged samples were adjusted to equal volume and resuspended in 2X Laemmli buffer (BioRad, Cat. #1610747) supplemented with 10% β-mercaptoethanol (MilliporeSigma, Cat. #M3148). Samples were boiled for 10 min, loaded on a 10% SDS-polyacrylamide gel, and processed as described above by immunoblot analysis. Single-cell imaging Overnight cultures were diluted 1:200 (or 1:100 for Δ bamD cultures due to their low cell density) and grown at 37 °C, followed by two 1:10 dilutions (at OD 600 around 0.1) to generate steady-state log-phase cells. Cells were imaged on a Nikon Eclipse Ti-E inverted fluorescence microscope with a 100X (NA 1.40) oil-immersion objective (Nikon Instruments). Images were collected on a Zyla 5.5 sCMOS camera (Andor Technology) using µManager v. 1.4 [37] . 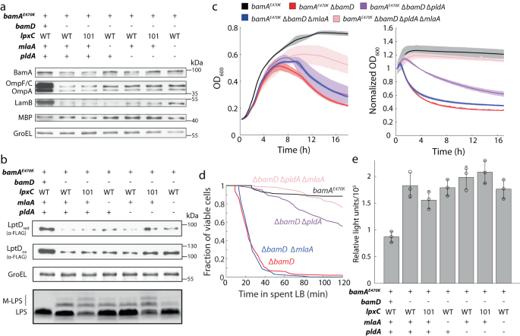Fig. 3: OM lysis is not due to loss of material but instead due to alteration in membrane composition. abamDdeletion reduces levels of OM proteins. Shown are immunoblots of major OM proteins in cell lysates ofbamAE470K, ΔbamD, and suppressor mutants of ΔbamDfrom log-phase cultures. Data are representative of three biological replicates.bAlthough deletion ofbamDreduces levels of the LPS transport protein LptD, LPS levels are unaffected. Shown are immunoblots of LptD, GroEL (as a control), and LPS in cell lysates ofbamAE470K, ΔbamD, and suppressor mutants of ΔbamDfrom log-phase cultures. Data are representative of three biological replicates.cThe decrease in OD in stationary phase (left) or upon transition from log-phase growth to spent LB (right, transition occurs att= 0) in ∆bamDcells is partially rescued by deletion ofpldAand fully rescued by deletion ofpldAandmlaA.N= 3 biological replicates. Curves are mean values, and shading represents 1 standard deviation.dCell lysis in spent LB is partially rescued by deletion ofpldAand almost fully rescued by deletion ofpldAandmlaA, in agreement with the population-level measurements in (c). Shown are quantifications of the fraction of viable cells as determined from time-lapse images (Methods).n> 100 cells for each strain.eSuppressors do not rescue the permeability defect of ∆bamDcells. Shown is quantification of the intake of fluorescent 1-N-phenyl-naphthylamine (NPN) inbamAE470K, ΔbamD, and suppressor mutants. Data are presented as mean values ± 1 standard deviation.N= 3 biological replicates. Relative light units = fluorescence/OD600. Cells were maintained at 37 °C during imaging with an active-control environmental chamber (HaisonTech). For single-cell imaging on agarose pads, 1 µL of cells was spotted onto a pad of 1% agarose in fresh LB. For microfluidic flow-cell experiments, including the spent medium assays, the oscillatory osmotic shock assays, and the plasmolysis/lysis assays, cells were loaded into CellASIC ONIX microfluidic flow cells (Sigma-Aldrich, Cat. #B04A-03-5PK) and medium was exchanged using the CellASIC ONIX2 microfluidic platform (Sigma-Aldrich, Cat. #CAX2-S0000). Imaging in microfluidic flow cells ONIX B04A plates were loaded with medium and pre-warmed to 37 °C. Exponentially growing cells were incubated at 37 °C in fresh LB without shaking for 60 min before transitioning into experimental conditions and imaging. For spent medium assays, cells were perfused with spent LB subsequent to fresh LB. For oscillatory osmotic shock assays, cells were subjected to alternating hyperosmotic shocks of 400 mM sorbitol (Sigma-Aldrich, Cat. #S1876, dissolved in LB) and recovery without sorbitol, with a period of 2 min (1 min shock and 1 min recovery). For plasmolysis/lysis assays to measure OM stiffness, cells were subjected first to hyperosmotic shock with 1 M sorbitol in LB and then treated with 5% N-lauroylsarcosine sodium salt (MP biomedicals, Cat. #190289) to remove the OM. Cells were stained with 300 µM 3-[[(7-Hydroxy-2-oxo-2H-1-benzopyran-3-yl)carbonyl]amino]-D-alanine hydrocholoride (HADA, MedChemExpress, Cat. #HY-131045/CS-0124027) and perfused with 0.85X PBS prior to the osmotic shock. Spheroplast induction Cells from a log-phase culture were loaded into an ONIX B04A plate and perfused with fresh LB and 2 µg/mL FM 4-64 (Invitrogen, Cat. #T13320) for 1 h, followed by 1 M sorbitol in LB for 10 min to induce plasmolysis. Plasmolyzed cells were treated with 1 mg/mL lysozyme (Sigma-Aldrich, Cat. #L6876) and 1 M sorbitol in LB to digest the cell wall, creating spheroplasts within 15 min of lysozyme treatment. Spheroplast cell contours were measured immediately after the loss of rod shape to minimize the impact of subsequent growth. Image analysis Time-lapse images were first segmented with the software DeepCell [38] , and the resulting segmented images were analyzed using Morphometrics [39] to obtain single-cell lineages and cell contours at sub-pixel resolution. Cell width and length were calculated using the MicrobeTracker meshing algorithm [40] . For plasmolysis/lysis assays, image segmentation and cell length measurements were performed using Morphometrics . Single-cell growth rate and morphology analysis The instantaneous growth rate of individual cells was computed using cell contour and cell lineage data obtained using Morphometrics . The two-dimensional projected cell area A was used as a proxy for cell biomass. At each time point, instantaneous growth rate was calculated from a local linear fit of ln( A ). We determined the longitudinal axis of each cell contour and measured local cell width at equally spaced locations along the longitudinal axis. 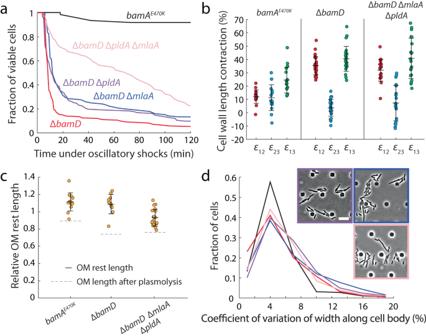Fig. 4: Replacement of proteins with PLs does not restore cell shape or OM stiffness. aLysis due to oscillatory hyperosmotic shocks (cycles of 1 min in LB and 1 min in LB + 400 mM sorbitol; Methods) is partially rescued by deletion of bothpldAandmlaA. Shown are measurements of the fraction of viable cells from time-lapse images in a microfluidic flow cell.n= 60 forbamAE470K;n> 100 cells for all other strains.bΔbamDand ΔbamDΔpldAΔmlaAcells have lower OM stiffness than the parent strain. Shown are measurements of cell wall length contraction from the turgid state to plasmolyzed state after addition of 1 M sorbitol (ε12), from the plasmolyzed state to lysed state after addition of detergent (ε23), and from the turgid state to the lysed state (ε13) (Methods). ε12and ε23are higher and lower, respectively, in ΔbamDand ΔbamDΔpldAΔmlaAcompared with the parent strain, suggesting that the OM in the two mutants is not as able to resist contraction upon turgor release. Data are presented as mean values ± 1 standard deviation. Sample sizes:n= 17 forbamAE470K,n= 24 for ΔbamD(plus 6 cells for ε12only),n= 20 for ΔbamDΔpldAΔmlaA.cThe OM rest length is similar to that of the turgid cell inbamAE470K, ΔbamD, and ΔbamDΔpldAΔmlaAcells, indicating that the OM of all strains have a similar amount of material. Shown is the ratio of the OM size of a spheroplast compared to the turgid OM area (Methods). In all three strains, the OM rest length is substantially larger than a cell after plasmolysis (ratio of OM length after plasmolysis to the turgid length is shown as grey dashed lines).N= 1 biological replicate. Data are presented as mean values ± 1 standard deviation. Sample sizes:n= 13 forbamAE470K,n= 11 for ΔbamD,n= 20 for ΔbamDΔpldAΔmlaA.dCell shape defects due tobamDdeletion are not rescued in the suppressor strains ΔbamDΔpldA, ΔbamDΔmlaA, and ΔbamDΔpldAΔmlaA. All three strains exhibited higher coefficient of variation in cell width along the cell body compared to the parent. Lines are colored by strain as in (a).n> 200 cells for each strain. Insets: cells were imaged during log-phase growth in a microfluidic flow cell. Scale bar: 10 µm. 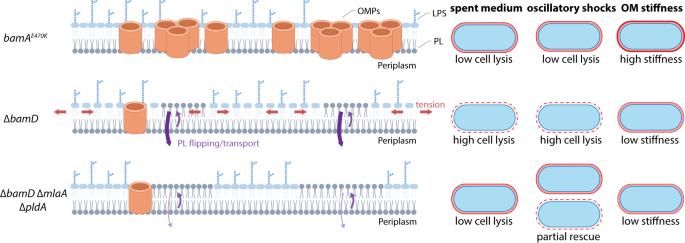Fig. 5: Model of OM destabilization by the severe reduction in protein content due tobamDdeletion. When ∆bamDcells are transferred from log-phase growth to spent LB or exposed to oscillatory osmotic shocks, they exhibit much higher rates of cell lysis than the parentbamAE470Kstrain, due to a reduction in OMP levels and consequent decrease in OM stiffness. Deletion ofmlaAandpldAincreases the amount of PLs in the outer leaflet of the OM, which relieves interleaflet tension and prevents lysis in spent medium. However, the ∆bamD∆mlaA∆pldAmutant exhibits only partial rescue of lysis under oscillatory osmotic shock and OM stiffness remains low. The coefficient of variation (CV) of cell width was defined for each cell as the ratio of the standard deviation to the mean of local width measurements along the rod-shaped cell body (measurements at the poles were excluded based on the curved geometry). Calculation of OM rest length and estimation of OM stiffness To calculate OM rest length, we used Morphometrics to measure HADA-labeled cell-envelope contours before and after plasmolysis and FM 4-64-labled OM contours of wall-less spheroplasts induced by lysozyme as described above. For each cell, we calculated the surface area of the turgid cell, A turgid , from its contour by assuming rotational symmetry around its long axis. After digestion of the cell wall by lysozyme, the OM adopted an amorphous shape, while remaining trapped in the flow cell with height assumed to be equal to the cell width before plasmolysis, w . We calculated the surface area of the OM, A OM , using its two-dimensional area, a , and contour length, s , via the relation A OM = 2 a + ws . Finally, to calculate the rest length of the OM, l OM , defined as the length of the OM if it were reshaped into a rod cell shape of width w , we used the equation l OM = l turgid + ( A OM − A turgid )/(π w ). Here, we approximated a rod-shaped cell as a cylinder capped by two hemispheres. Thus, the difference between the length of a turgid cell and the OM rest length is proportional to the difference between the corresponding surface areas by a factor of 1/(π w ), the reciprocal of the cross-sectional perimeter. OM stiffness was estimated using a plasmolysis-lysis assay [3] performed in a CellASIC ONIX microfluidic flow cell (Sigma-Aldrich, Cat. #B04A-03-5PK). Cell length was measured in the turgid state ( l 1 ), under plasmolysis ( l 2 ), and after lysis ( l 3 ). Length contractions between these states were calculated as ε 12 = ( l 1 − l 2 )/ l 2 , ε 23 = ( l 2 − l 3 )/ l 3 , and ε 13 = ( l 1 − l 3 )/ l 3 . The OM stiffness k OM relative to that of the cell wall k CW was estimated using the average value of the length contractions as k OM = k CW <ε 23 >/[<ε 12 > (1 + <ε 23 >)], as in ref. [3] . Reporting summary Further information on research design is available in the Nature Portfolio Reporting Summary linked to this article.